Dynamically self-assembled silver nanoparticles as a thermally tunable metamaterial The availability of metamaterials with properties that can be actively tuned is crucial for the future development of various metamaterial-based technologies. Here we show that by using silver nanoparticles equipped with a thermally responsive organic coating a metamaterial is obtained with reversibly switchable properties. The material investigated exhibits dynamic self-assembly resulting from temperature-dependent changes of organic coating shape, which translates to a switchable spatial distribution of the silver nanoparticles. This in turn strongly influences the optical properties of the entire material. The measured optical characteristics of the material are in excellent agreement with theoretical calculations, which allow us to use the latter to predict a dynamically tunable epsilon-near-zero behaviour of the metamaterial. The suggested methodology opens new routes for tunable metamaterials that operate in the visible region and will enable various applications for soft-matter-based optical devices. Self-assembly (SA) of nanoparticles (NPs) into ordered structures is a formidable challenge in many branches of material science, especially for metamaterials research [1] , [2] , [3] , [4] . Beyond being fascinating from an intellectual perspective, self-assembled metamaterials provide a clear solution to some open problems that have to be solved before metamaterials can evolve to a mature technology. This especially concerns the availability of metamaterials in large-scale quantities and as bulk materials. To date, SA of NPs provided access to materials exhibiting topological darkness [5] , epsilon-near-zero (ENZ) behaviour [6] , [7] , [8] , magnetic-based Fano resonance scattering at optical frequencies [9] , efficient absorbance properties [10] and also enabled optical cloaking [11] , [12] . However, the established SA approaches to form metamaterials result in static structures. This severely limits their functionality since metamaterials with tunable characteristics are often required for many budding applications [13] , [14] , [15] , [16] , [17] , [18] , [19] , [20] , [21] . Various approaches have been explored to achieve dynamically reconfigurable metamaterials, including embedded varactors [22] , metamaterial hybridization with liquid crystals [21] , [23] , the use of electromechanical [20] , elasto-electromagnetic [17] and laser-induced [18] modulation as well as exploitation of phase-change materials [14] , [15] , [16] . However, dimensions of these structures are usually on the order of μm or hundreds of nm, which results in operation wavelengths outside the visible region, highlighting the need for tunable metamaterials made of nanocrystal solids. To this end, broad tunability of nanocrystal solids’ properties has been achieved, for example, by marked decreasing interparticle spacing, which enhances interparticle coupling. Potentially the best developed strategy of this kind is based on exchange of large, organic ligands that are usually used in the nanocrystals synthetic process to small inorganic molecules [24] , [25] , [26] , [27] . Some conspicuous examples of application of this approach include switching insulating PbSe nanocrystal arrays to an n-type semiconductor [28] and dielectric-to-metal transition of Au NPs aggregates [2] . However, these changes are predominantly irreversible, whereas active tunability of properties is necessary to achieve tunable metamaterials. Those limitations may be overcome by using dynamic SA (DSA) of NPs. DSA would unlock the opportunities of an active engineering of aggregate structures and associated properties as lately evidenced by theoretical modelling [29] , [30] . Recently, a handful of DSA methods have been reported [31] , [32] , [33] , [34] , but most of these techniques rely unfortunately on solvated environments, which result in very low NP-filling fractions, or are limited to two-dimensional systems [35] , [36] . Therefore, the application of these methods in metamaterials research is limited. It would be of utmost importance to obtain large metal-filling fractions to access materials that deviate from weakly dispersive dielectric properties exhibited by strongly diluted metallic NP arrays. Devising new DSA strategies to obtain reconfigurable, densely packed NP assemblies is therefore of paramount importance. Notably, DSA of metal particles is a complementary approach to the use of static SA of nanocrystals made of phase-change material, which was recently reported [13] . Both provide access to reversible, thermally switchable metamaterials and underline the surge for tunable metamaterials based on NPs. Here, we show that DSA of NPs can lead to a system with theoretically predicted tunable metamaterial properties. To achieve this we used a SA strategy based on liquid-crystalline (LC) surface ligands. Recently, this approach has been intensively explored for both non-plasmonic and plasmonic NPs [37] , [38] , [39] , [40] , [41] , [42] , [43] , [44] , [45] . Also, this strategy was shown to enable the formation of dynamic assemblies [46] , [47] . For example, Wojcik et al . [47] prepared a gold NP aggregate, which exhibited structural polymorphism—lamellar, rectangular, columnar and hexagonal phases were identified for a single sample at various temperatures. A LC strategy to DSA was also used by Umadevi et al . [46] to create magneto-responsive materials made of LC-coated gold nanorods, in which spatial orientation of the rods was changed with a handheld magnet. However, in none of these systems were optical properties of the assemblies investigated. Another strategy for achieving DSA of NPs into dense arrays is using polymer nanocomposites [48] , [49] , [50] . Unfortunately, this strategy suffers from the complexity of achieving initial dispersion of NPs, low NP loadings [51] and usually collective interactions of NPs were not examined. Only lately, chiral plasmonic DNA nanostructures with switchable circular dichroism [52] , and switchable dispersion of Au NPs with reversible tunability of the aggregate optical characteristic were obtained [50] . Plasmonic band shifting by 5 nm was observed in the latter report after thermal annealing of the material for tens of minutes. However, from the applicative point of view it would be advisable to improve two parameters of such systems—enhance kinetics of the optical tunability and broaden the range of the optical response [53] . Herein, we report the synthesis of a dense Ag NP aggregate that undergoes heat-induced, reversible spatial reconfiguration from lamellar to the isotropic phase. Notably, this reorganization results in NP nearest-neighbour distance variation allowing active engineering of collective interactions between NPs. The relatively large separation between nanocrystals assured by organic coating does not allow us to observe marked changes of properties, for which achieving smaller interparticle gaps is necessary, therefore the expected tunability is limited to the strongly dispersive dielectric regime. The switching behaviour is evidenced by shifting of the aggregate plasmon band maxima position. We achieve tunability in the range of up to 20 nm for slow cooling and heating (tens of minutes). We also present the possibility of fast switching (ten of seconds) but with slightly lower optical response—14-nm shift. Importantly, the DSA methodology presented here allows continuous tunability of plasmonic properties, in contrast to most of DSA methods reported to date, which usually allow only switching between on and off states of the collective interactions. To fully confirm that the optical response of our material emerges from structural reorganization of NPs, we calculate extinction spectra of the aggregate obtained by slow cooling/heating using full-wave electromagnetic simulation tools, and found the modelled spectra to be in excellent agreement with the experiment. This numerical analysis also provides insight into metamaterial properties of the slowly switched system, indicating tunable ENZ behaviour. ENZ properties are further confirmed by ellipsometric measurements, which enable us to extract effective optical properties of the system. Lately, ENZ materials attract considerable interest, since they allow for precise phase manipulation of light [54] , [55] , [56] . ENZ materials based on nanocrystal solids that enable guiding and confining signals on the nanometre scale are especially interesting. Also, they can be designed to work in the entire visible spectrum [57] , which is indispensable for future optical fibre and optical computing technologies. In contrast to static examples of such materials [6] , [7] , [8] , here we report a NP-based material that exhibits theoretically predicted tunable ENZ properties enabling broadband function. Design and synthesis of hybrid NPs To construct a tunable NP aggregate with likely metamaterial properties, we have synthesized LC-coated silver NPs following a two-step procedure shown in Fig. 1 (refs 21 , 35 ). First, ca. 4.7±0.5-nm diameter (as determined with transmission electron microscopy (TEM), Fig. 1a ) dodecanethiol-coated silver NPs were obtained using a previously reported [38] modification of the Wang procedure [58] . Then, in a ligand-exchange reaction, a promesogenic molecule (L, Fig. 1b , details of the synthesis are given in Methods, Supplementary Note 1 and Supplementary Fig. 1 ) was introduced into the NP surface, yielding hybrid silver NPs (Ag@L, Fig. 1c ). The ligand-exchange reaction did not affect mean diameter of NPs but slightly increased metallic core size distribution (4.7±0.6 nm; as determined with TEM). It should be noticed that the free compound L does not form LC phases and melts directly into the isotropic phase at ~87 °C, but mesogenic properties of the ligand are not prerequisite for inducing SA of NPs into the LC phase [59] , [60] . Also, molecules with similar architecture to L, comprising three aromatic rings with ester linkages, were reported to support formation of LC phases [61] . Therefore, L can be viewed as a promesogenic structure in which a small change of substituents would result in LC properties. Terminal groups of the promesogenic molecule were chosen based on our previous experience with LC-NPs [38] , [59] —hexadecyloxy chain was used to provide fluidity to the hybrid system, while a 15-carbon-length mercapto-functionalized alkyl chain assured flexibility of the ligand and served as a docking moiety to the NP surface. To evaluate the chemical nature of Ag@L NPs, X-ray photoelectron spectroscopy (XPS) and wide-angle X-ray diffraction were used (see Supplementary Figs 2 and 3 , respectively). Wide-angle X-ray diffraction confirmed that metallic cores of NPs are composed of silver (cubic structure). XPS revealed the presence of expected atoms in the sample: silver, sulfur, carbon, oxygen and silicon (coming from the substrate) and allowed for quantitative elemental analysis (see details in Methods), confirming successful synthesis. The exact composition of the organic coating of A@L NPs was determined based on thermogravimetric analysis (TGA; see Supplementary Fig. 4 ) as described previously [38] . The organic shell of Ag@L is composed of ca. 240 alkane thiols and 260 L molecules, which in total is close to the number of alkanethiol ligands (520) grafted on the NP before the ligand-exchange reaction. 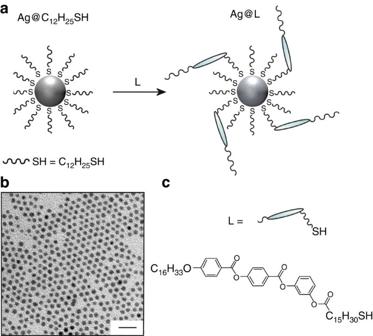Figure 1: Design and synthesis of hybrid Ag@L nanoparticles. (a) Scheme ligand-exchange reaction on dodecanethiol-coated Ag NPs (Ag@C12H25SH) leading to the hybrid material Ag@L. (b) TEM image of Ag@C12H25SH nanoparticles, scale bar, 20 nm. (c) Molecular structure of the promesogenic ligand L. Figure 1: Design and synthesis of hybrid Ag@L nanoparticles. ( a ) Scheme ligand-exchange reaction on dodecanethiol-coated Ag NPs (Ag@C 12 H 25 SH) leading to the hybrid material Ag@L. ( b ) TEM image of Ag@C 12 H 25 SH nanoparticles, scale bar, 20 nm. ( c ) Molecular structure of the promesogenic ligand L. Full size image Switching material structure To investigate SA properties of Ag@L NPs, we have used temperature-dependent small-angle X-ray diffraction (SAXRD) measurements and TEM imaging ( Fig. 2 ). For SAXRD a small portion of the Ag@L solution was dropcasted onto kapton foil and heated. At elevated temperatures (above 100 °C) a single, diffuse signal corresponding to the mean interparticle distance of ca. 7.2 nm was observed (as measured at 120 °C, Fig. 2a ), evidencing isotropic distribution of metallic cores within the sample—this structure will be referred to as the Iso phase. Subsequent lowering of the sample temperature resulted in a distinctive change of the diffraction pattern—three narrower Bragg scattering rings appeared, evidencing development of a long-range-ordered structure ( Fig. 2b ), resembling a LC lamellar structure. In this structure, metallic cores would form layers with well-developed interlayer distance of ca. 8.4 nm and interparticle (center-to-center) distance within the layer ca. 6.1 nm (as measured at 30 °C). For unambiguous determination of the structure we have attempted to prepare a monodomain sample by shearing the dropcasted Ag@L NPs at 50 °C. SAXRD measurements of the shear-aligned sample (see Supplementary Fig. 5 ) revealed two orthogonal signals indexed as (10) and (01), which are characteristic to a lamellar phase [38] , [59] , [62] and confirm the initial structure assignment. On the basis of the broadness of the (01) signal, we assume that the metallic cores of NPs are arranged on a rectangular lattice within the layer, although hexagonal packing is another possibility. This low-temperature structure will be referred to as Lm. It should be noted that the Lm phase is no typical liquid-crystal, since it does not show optical birefringence. SAXRD measurements alone provide a proof of DSA properties of hybrid NPs, since reversible switching between the two states of the aggregate, Lm and Iso, was possible by varying the temperature between 30 and 120 °C. The kinetics of the process will be discussed later, when considering optical properties of the material. 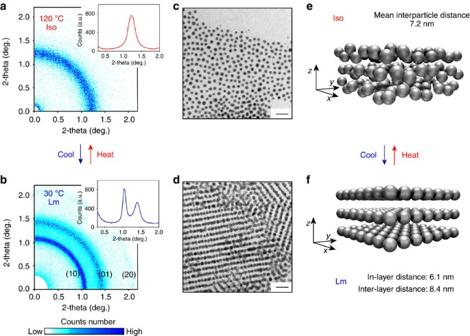Figure 2: Structural analysis of Ag@L aggregate switching. (a) Representative SAXRD image of Ag@L aggregate at elevated (120 °C) and (b) low (30 °C) temperatures, corresponding to isotropic (Iso) and lamellar (Lm) arrangements, respectively; colour intensity map of count number is given below; insets show one-dimensional scans of the diffractograms. (c) Representative TEM image of thermally annealed Ag@L nanoparticles revealing patterns corresponding to the Iso and (d) Lm structures, scale bar, 20 nm. (e) Scheme of nanoparticle arrangements in Iso and (f) Lm structures as deduced from SAXRD and TEM; organic ligands are omitted for clarity. Figure 2: Structural analysis of Ag@L aggregate switching. ( a ) Representative SAXRD image of Ag@L aggregate at elevated (120 °C) and ( b ) low (30 °C) temperatures, corresponding to isotropic (Iso) and lamellar (Lm) arrangements, respectively; colour intensity map of count number is given below; insets show one-dimensional scans of the diffractograms. ( c ) Representative TEM image of thermally annealed Ag@L nanoparticles revealing patterns corresponding to the Iso and ( d ) Lm structures, scale bar, 20 nm. ( e ) Scheme of nanoparticle arrangements in Iso and ( f ) Lm structures as deduced from SAXRD and TEM; organic ligands are omitted for clarity. Full size image To further confirm the above structural analysis we have turned to TEM imaging. Hybrid NPs were dropcasted onto a TEM grid that was subsequently heated to 120 °C and cooled instantly by removing from a heating stage. Regions corresponding to both Iso ( Fig. 2c ) and Lm ( Fig. 2d ) arrangements of NP metallic cores were found with interparticle distances almost identical to those derived from SAXRD; for the Lm phase, the measured interlayer distance was 8.5±0.4 nm, while for Iso the interparticle distance was 7.3±0.8 nm. By combining SAXRD and TEM results we were able to propose a model of the spatial arrangement of the Ag@L NPs cores ( Fig. 2e,f ) and consequently translate it into the organic corona shape. In the Iso phase, both promesogenic and alkyl ligands are evenly distributed in space forming a spherical entity, while in the Sm structure L molecules are mainly located in between the layers, and only partially contribute to the spacing within the layer. It is therefore the rearrangement of promesogenic ligands that causes the spatial rearrangement of NPs’ metallic cores. This behaviour has been previously observed for smaller gold NPs [59] , [62] and can be viewed as experimental realization of theoretically predicted DSA of shape-shifting particles [63] . 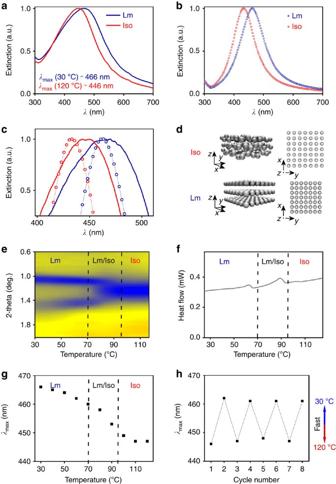Figure 3: Optical characterization of Ag@L aggregate. (a) Extinction spectra of the aggregate taken at 30 and 120 °C revealing a shift of plasmon band maxima (λmax). (b) Simulated extinction spectra of Lm and Iso structures. (c) Overlay of simulated and experimental extinction spectra. (d) Sketch of part of Iso and Lm aggregates (in fact layers comprised 17 × 17 particles) used in simulations. (e) Temperature-dependent SAXRD reflections evidencing regions of Lm, Lm/Iso and Iso structures’ existence (divided by the dashed lines), collected on heating with a 10-deg. step. (f) DSC trace, collected on heating, of hybrid nanoparticles. Phase transition region in which Lm/Iso structures coexist is between the dashed lines. (g) Temperature-dependentλmaxposition shift, corresponding to the structural reconfiguration shown ine. Phase transition region, as deduced based one, is between the dashed lines. (h) Reversible shifting ofλmaxposition in consecutive fast heating/cooling cycles. Switching material plasmonic properties Figure 3 shows the dynamic optical characteristic of the Ag@L NP aggregate. Ultraviolet–visible absorption measurements (see details in Methods) revealed a 20-nm blue shift, from 466 to 446 nm, of the plasmonic band ( λ max ) when the LC-NP aggregate was heated from 30 to 120 °C ( Fig. 3a ), which is for the aggregate reconfiguring from the Lm to Iso phase. To confirm that the shift originates from spatial redistribution of metal particles, absorption spectra of the NP assemblies were simulated using a multi-sphere scattering algorithm. The simulation was done with a program that solves self-consistently Maxwell’s equations for an arbitrary arrangement of a finite number of spheres for a given illumination. This is achieved by expanding the incident, the scattered and the internal fields of each sphere into eigenmodes. The amplitudes of all eigenmodes can be calculated by enforcing the usual boundary conditions at the surface of the spheres. All further properties can be derived from these coefficients. To consider the actual structure in the simulations, the Lm phase was built from three layers composed of 17 × 17 metal particles with spacing as derived from SAXRD measurements, while the Iso structure was approximated by randomly shifting NP positions of the Lm structure to reach a mean nearest-neighbour distance of 7.2 nm according to the measurements ( Fig. 3d ). In preliminary simulations it was carefully verified that this number of silver spheres is fully sufficient to reflect the properties of an infinite sample, that is, all quantities of interest converged. The organic corona of NPs was treated as a homogenous medium with a refractive index of 1.6, an intermediate value for LC molecules. A blue shift of λ max was retrieved form the simulations of the optical spectra from 463 to 438 nm ( Fig. 3b ). This is slightly larger than the measured values, but nevertheless the wavelengths of plasmonic bands’ maxima are in very good agreement with the experiment considering the complexity of the material ( Fig. 3c ). It is worth noting that for a structure similar to the Iso phase but with interparticle spacing corresponding to the nearest-neighbour distance in the Lm aggregate (6.1 nm), the retrieved λ max was almost identical to the one for the Lm structure. This shall evidence that the nearest-neighbour distance variation between the Lm and Iso structures is the crucial parameter influencing plasmonic band position. This conclusion is further supported with a control experiment—no shift of plasmonic band position was observed for a heated sample of dodecanethiol-coated silver NPs (see Supplementary Fig. 6 ), for which no structural reconfiguration is observed within the given temperature limit. Figure 3: Optical characterization of Ag@L aggregate. ( a ) Extinction spectra of the aggregate taken at 30 and 120 °C revealing a shift of plasmon band maxima ( λ max ). ( b ) Simulated extinction spectra of Lm and Iso structures. ( c ) Overlay of simulated and experimental extinction spectra. ( d ) Sketch of part of Iso and Lm aggregates (in fact layers comprised 17 × 17 particles) used in simulations. ( e ) Temperature-dependent SAXRD reflections evidencing regions of Lm, Lm/Iso and Iso structures’ existence (divided by the dashed lines), collected on heating with a 10-deg. step. ( f ) DSC trace, collected on heating, of hybrid nanoparticles. Phase transition region in which Lm/Iso structures coexist is between the dashed lines. ( g ) Temperature-dependent λ max position shift, corresponding to the structural reconfiguration shown in e . Phase transition region, as deduced based on e , is between the dashed lines. ( h ) Reversible shifting of λ max position in consecutive fast heating/cooling cycles. Full size image To get a more precise picture of the influence of the spatial distribution of the NPs metallic cores on λ max , we have performed structural and optical measurements of Ag@L NPs heated in a stepwise manner (data collected every 10 °C, on heating, Fig. 3e,g ). Up to 70 °C, the Sm phase is solely observed as evidenced by SAXRD but heating causes an expansion of the NP gap within the layers, while the interlayer distance reduces. This behaviour translates to a slow shift of λ max towards smaller values. Then, in between 70 and 95 °C a phase transition is observed from Lm to Iso phase—both structures coexist within this temperature range. The phase transition is accompanied with a faster kinetics of λ max blue shift. Finally, above 95 °C the Iso phase is solely found and the plasmonic band maximum reaches the lowest wavelength. Evaluation of the switching mechanism To understand the behaviour of promesogenic ligands during the heating process, we have performed DSC measurements of hybrid NPs with a heating rate of 5 deg. min −1 ( Fig. 3f ). Two evident thermal events were identified taking place at ca. 60 and 90 °C. When compared with SAXRD results, it can be noticed that the first event can be associated with sharpening of the Bragg signal showing in-layer distance between NPs. Likewise, the second corresponds to the transition from Lm to Iso structure. It is therefore the melting of L molecules at ca. 90 °C that causes a rearrangement of silver NPs’ metallic cores. Kinetics and reversibility of switching Next, we investigated the reversibility of Ag@L aggregate reconfiguration and examined the impact of the kinetics of temperature variation on the process. Both these parameters are important from the point of view of DSA and future applications. Noticeably, both structural and optical properties are fully reversible as attested by SAXRD and ultraviolet–visible measurements, but for this purpose slow cooling is needed. A well-developed Lm structure can be achieved by changing the temperature from 120 to 30 °C in a stepwise manner with a 10 °C step, which takes ca. 60 min. Iso phase can be accessed more easily, still incubation in 120 °C for few minutes is necessary to achieve the maximum plasmonic band shift. It would be advantageous to achieve fast switching behaviour; therefore, we tested the optical response of the sample to heating/cooling cycles lasting only tens of seconds. SAXRD measurements of Ag@L aggregates cooled fast revealed coexistence of Lm and Iso phases ( Supplementary Fig. 7 ). This translates to a lowered magnitude of plasmonic band shift in comparison with slow kinetics of cooling; a mean λ max variation of ca. 14 nm was observed when the sample was quickly cycled between 120 and 30 °C ( Fig. 3h ). Importantly, on the short term the tested hybrid NPs do not undergo decomposition at elevated temperatures as evidenced by 1H nuclear magnetic resonance (NMR) investigation ( Supplementary Fig. 8 ); however, on the long term the system would probably slowly decompose due to oxidation of surface silver atoms [54] causing release of stabilizing surface ligands. Modelling metamaterial properties The properties of the Ag@L NP aggregate were then considered in respect of achieving an ENZ regime. The effective dielectric function ( ε eff ) was calculated for Iso and Lm phases ( Fig. 4a,b ). The Clausius–Mossotti relation was used considering a particle in a lattice with the appropriate filling fraction corresponding to the respective interparticle distances. For the lamellar aggregate we used a second method, retrieving the effective properties from the complex reflection and transmission coefficients calculated assuming an infinitely extended rectangular lattice. We found very good agreement with the result from the Clausius–Mossotti relation. In both cases, the real part of ε eff exhibits both positive and negative regions due to a strong Lorentzian resonance centred at the collective surface plasmon polariton resonance. Such properties are characteristic to transparent and metallic materials, respectively. Importantly, the real part of the permittivity reaches zero, allowing us to classify this material as ENZ, for Lm and Iso structures at slightly different wavelengths. For an actual application, the short-wavelength regime is very likely attractive since it is off-resonant and propagating light would therefore experience lower absorption. It should be also noted that, for modelling purposes small monodomains of Lm and Iso aggregates are considered. This should be fully sufficient to describe the global arrangement properties, since the monodomains are optically comparable and no non-local effective properties are observed in the process of homogenization. This strongly supports the idea that the material is an actively tunable metamaterial. 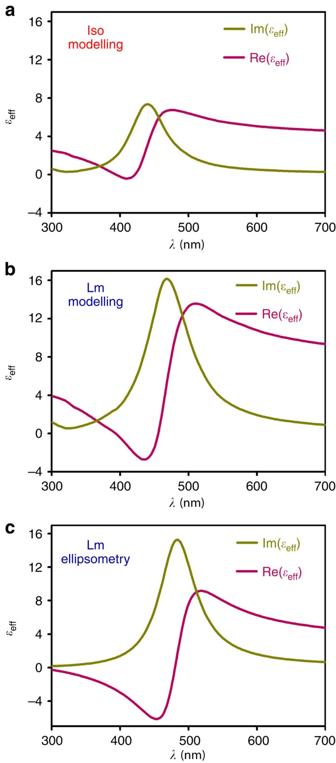Figure 4: Epsilon-near-zero properties of Ag@L material. (a) Theoretically predicted imaginary (Im(εeff)) and real (Re(εeff)) parts of the dielectric function of Ag NP aggregates in the Iso and (b) Lm structure. (c) Dielectric functions calculated based on spectroscopic ellipsometry measurements. Figure 4: Epsilon-near-zero properties of Ag@L material. ( a ) Theoretically predicted imaginary (Im( ε eff )) and real (Re( ε eff )) parts of the dielectric function of Ag NP aggregates in the Iso and ( b ) Lm structure. ( c ) Dielectric functions calculated based on spectroscopic ellipsometry measurements. Full size image To determine the bandwidths of the ENZ properties of the Ag@L material in the Lm and Iso phases, various criteria can be considered as introduced previously by other authors [8] , [54] , [64] , [65] . Rough estimation, for example, based on identifying the spectral range where Re( ε eff ) values are in between −1.0 and 1.0 yields ENZ properties for wavelengths’ ranges 365–410 nm for Lm, and 375–430 nm for Iso structures ( Supplementary Fig. 9 ) [8] , [54] . Naturally, narrower ENZ regions are retrieved if Re( ε eff ) values are restricted to the −0.2 to 0.2 range as used by Pinchuk et al . [64] , yet tunability is still observed ( Supplementary Fig. 9 ). Obviously, the real part of the permittivity is exactly equal to zero only at a single wavelength. We wish to stress that the effect we exploit is resonant, which means that dispersion is always accompanied by absorption. Although we work at off-resonant frequencies, absorption remains notable. Following suggestions from literature [65] , we quantify this influence using a figure of merit (FOM) defined according to equation (1): Equation (1) expresses the propagation length of light in the ENZ material in units of the wavelength. Using the permittivity values retrieved from the simulations a FOM of ~0.5 is found at the wavelength where the real part of epsilon is zero. In the ENZ window of the Lm structure (365–410 nm), the propagation length of light takes values between 0.4 and 1.2 wavelengths. For the Iso structure the extreme values of FOM in the ENZ region are 0.4 and 1.0. To further confirm ENZ properties of the NP assembly, we have performed variable wavelength ellipsometric spectroscopy of a thin film of Ag@L material on a silicone substrate (details of the measurements are given in the Methods). Prior to the measurements the material was thermally annealed to assure Lm arrangement of NPs and the thickness of the film was measured using atomic force microscopy (AFM) ( Supplementary Fig. 10 ). For the purpose of fitting the acquired ellipsometric data (amplitude and phase of reflected light versus light wavelength, Supplementary Fig. 11 ), we rely on a complex function for the effective permittivity based on two assumptions—that the material is made from small, spherical particles made of silver (properties of which can be reflected by a permittivity function for Ag that is built in the software) embedded into an organic matter with aromatic moieties (properties thereof are reflected by a harmonic oscillator with free parameters). It should be noted that similar results were obtained when using an effective medium approach with Bruggeman analysis, approximating the medium as a mixture of aromatic molecules (reflected by an oscillator) and silver (reflected by the built-in permittivity for Ag) [2] , [64] . Similar approaches have been applied successfully in the past to describe effective properties of composites with a comparable topography [2] . The outlined procedure enabled us to retrieve macroscopic, dielectric functions of the Ag@L sample having Lm order ( Fig. 4c , for real and imaginary parts of refractive index see Supplementary Fig. 12 ), which are in very good agreement with the theoretically predicted properties. In the outlined paper we have achieved DSA of silver NPs for which metamaterial properties were simulated and verified by ellipsometry measurements. LC ligands grafted onto the metallic surface were used to drive the reconfiguration of the aggregate from a lamellar to an isotropic structure. Variation of spatial distribution of NPs allows engineering the nearest-neighbour interparticle gap in the 2.5–1.4-nm range and results from the changes of the geometry of the organic coating layer. This translates to switching of the aggregate plasmonic band position by 20 nm and allows active tunability of the materials dielectric functions. Notably, the relatively thick organic coating results in a metal volume fraction suited for the observation of ENZ properties. The ENZ properties are observed for wavelengths in between 365 and 430 nm, which is especially interesting due to the need for metamaterials working in the visible range for future optical electronics technologies. Importantly, the spectral regions for Iso and Lm structures are slightly different, confirming tunability of the metamaterial properties. Another key feature of the presented system is that the observed switching behaviour of the material is fully reversible both in the view of structure and properties if slow cooling is used. Fast changes of temperature also result in a change of the optical response but with a slightly decreased magnitude of the plasmonic band shift. The approach to reconfigurable metamaterials presented here provides opportunities, but it also puts some challenges. The range of the tunability is limited due to the use of large surface ligands, therefore profound changes of the physicochemical characteristic (for example, dielectric-to-metal transition) of the material can hardly be achieved since interparticle gaps smaller than 0.5 nm are necessary to assure strong interparticle coupling. This problem can be addressed either by minimizing the lowest interparticle gap or assembling larger silver particles, keeping the thickness of the organic coating constant. Achieving these goals would be non-trivial, however, it should be noted that both unusually low interparticle spacing [37] (ca. 1 nm) and assembly of larger NPs [40] (ca. 10 nm) using the outlined strategy have been reported. Proper design of surface ligands should also allow to lower the phase transition temperature, assuring long-term stability of the material. The final challenge is kinetics of the reconfiguration. The current state-of-the-art are switching times on the scale of microseconds achieved by Zheludev et al . [20] , which are beyond the scope of our approach. The presented material allows for reconfiguration on the scale of tens of seconds, comparable to other systems based on DSA of nanocrystals; however, the use of liquid crystals as the driving force for rearrangement allows one to predict that tunability on shorter timescales will be achievable. In summary, the strategy presented here achieves tunability of a NP aggregate with ENZ properties evidencing that next-generation materials with adaptive behaviour can be obtained via the LC approach. Materials and equipment Solvents and substrates were obtained from Sigma-Aldrich. Before use solvents were dried over activated molecular sieves for 24 h. Substrates were used without further purification. All reactions were carried out under nitrogen (N 2 ) atmosphere in dried glassware and assuring efficient magnetic stirring. Purification of reaction products was carried out by column chromatography using RushanTaiyang silica gel 60 (230–400 mesh) at atmospheric pressure or by crystallization if possible. Analytical thin-layer chromatography was performed using a Silica Gel 60 Å F254 (Merck) pre-coated glass plater (0.25 mm thickness) and visualized using iodine vapour and/or an ultraviolet lamp (254 nm). Yields refer to chromatographically and spectroscopically ( 1 H NMR) homogeneous materials. The 1 H NMR and 13 C NMR spectra were recorded at either 200 or 500 MHz NMR Varian Unity Plus. Proton chemical shifts are reported in p.p.m. ( δ ) relative to the internal standard—tetramethylsilane (δ=0.00 p.p.m.). Carbon chemical shifts are reported in p.p.m. ( δ ) relative to the residual solvent signal (CDCl 3 , δ =77.0 p.p.m.). Data are presented as follows: chemical shift, integration, multiplicity (s=singlet, d=doublet, t=triplet, q=quartet, br=broad and m=multiplet), and coupling constant (Hz). In all recorded spectra there are also sharp signals coming from a small amount of known impurities present in used solvent: H 2 O (1.7 p.p.m.) and CHCl 3 (7.27 p.p.m.). SAXRD patterns for the powder as well as partially aligned samples were obtained with the BrukerNanostar system. The CuKα radiation was used; patterns were registered with an area detector VANTEC2000. The temperature of the sample was controlled with a precision of 0.1 K. Kapton tape was used as a substrate for NP measurements. XPS experiments were performed in a PHl 5,000 VersaProbe—Scanning ESCA microprobe (ULVAC-PHI, Japan/USA) instrument at a base pressure below 5 × 10 −9 mbar. Monochromatic Al Kα radiation was used and the X-ray beam, focused to a diameter of 100 μm, was scanned on a 250 × 250-μm surface, at an operating power of 25 W. Photoelectron survey spectra were acquired using a hemispherical analyzer at pass energy 117.4 eV with a 0.4-eV energy step; core-level spectra were acquired at pass energy 23.5 eV with a 0.1-eV energy step. All spectra were acquired with 90° between X-ray source and analyzer and with the use of low-energy electrons and low-energy argon ions for charge neutralization. After subtraction of the Shirley-type background, the core-level spectra were decomposed into their components with mixed Gaussian–Lorentzian (30:70) shape lines using the CasaXPS software. Quantification calculations were conducted using sensitivity factors supplied by PHI. Spectra were calibrated against 284.6 eV for C 1 s region. Transmission electron micrography was performed using a Zeiss Libra 120 microscope, with LaB6 cathode, equipped with OMEGA internal columnar filters and a charge-coupled device camera. TGA were performed with a TA Q50 V20.13 (TA Instruments) analyzer. The measurements were carried out in the 20–600-°C range with 10 K min −1 heating rate in air. The ultraviolet–visible spectrum was measured using a Cary 5,000 spectrometer (Agilent). The solutions of functionalized particles in dichloromethane were held in standard poly(methyl methacrylate) (PMMA) cuvettes (VWR) with a 10-mm optical path, while the aggregates were recorded on a quartz substrate in a transmission mode. TEM images were taken using the Zeiss Libra 120 microscope. Ellipsometric measurements were made using a variable-angle spectroscopic ellipsometer SENTECH SE850 (SENTECH Instruments GmbH). The acquired data were analysed using SpectraRay II software package. AFM measurements were performed in tapping mode with a Dimension Icon (Bruker) microscope using SCANASYST-AIR tip (silicon tip on nitride lever). NP synthesis Silver clusters with dodecanethiol coating were prepared as previously described [25] using a modified literature method [37] . Fifty ml of dodecylamine (1.5 g) solution in cyclohexane (50 ml) was stirred for 10 min with 12 ml aqueous formaldehyde (37%). The organic phase was separated out and washed twice with water (2 × 50 ml). Then, aqueous solution of AgNO 3 (0.4 g AgNO 3 in 20 ml H 2 O) was added, left to stir for 40 min after which dodecanethiol (0.3 molar eq. of dodecylamine) was added and the reaction was stirred overnight. Organic phase was separated and NPs were precipitated by addition of 100 ml of ethanol. The precipitate was centrifuged, collected, dissolved in a small amount of cyclohexane (10 ml) and again the precipitation procedure was repeated. The obtained NPs (Ag@C 12 H 25 SH) were used as the starting material for the preparation of hybrid NPs, denoted as Ag@L. To 15 mg of NPs dissolved in 10 ml hexane/dichloromethane (DCM) mixture ( v / v =1/1) 20 mg of the L ligand was added. The reaction proceeded at room temperature for 24 h. Then, NPs were precipitated with 20 ml of methanol and centrifuged (13,000 r.p.m., 5 min). Supernatant containing unbound thiol ligands was discarded. The precipitate was dissolved in 1 ml of warm hexane and centrifuged after cooling down; then, the process was repeated. This washing procedure was repeated until no traces of free mesogenic ligand remained, as determined by thin-layer chromatography. Thermogravimetric analysis of NPs To evaluate the exact composition of organic coronas of the studied NPs, TGA was used. The weight loss for dodecanethiol-coated silver NPs (Ag@C 12 H 25 SH, below 260 °C) was 23.40%. This value was attributed to the removal of the organic shell and recalculated to the number of surface alkyl thiols as outlined below. TGA traces for hybrid NPs (Ag@L) revealed substantially larger weight losses in two distinct steps. The first one, below 260 °C can be attributed to the removal of alkyl thiol molecules and accounts for a mass drop of 12%. A wider peak at higher temperature values (>260 °C) is due to the removal of L molecules (weight loss 35.37%). The numbers of alkyl ( N alkyl ) and mesogenic ligands ( N L ) were calculated as given below. To convert the mass loss measured by the TGA measurements to surface ligand stoichiometry, we first calculated the mass of single metal spheres for silver ( M Ag ) NPs, using the diameter derived from SAXS and TEM and the bulk density of metals ρ Ag =10.49 g cm −3 . The calculated mass was: M Ag =5.7 × 10 −19 g. The mass of organic matter ( M org ) removed from a single NP was calculated using % of mass left after the analysis (% M left ) and % of mass loss (% M loss ) using equation (2): can be read out of Supplementary Fig. 4a . To retrieve the number of ligands per NP, M org has to be divided by the mass (in (g)) of the ligand responsible for the given mass drop: m C12H25SH =3.36 × 10 −22 g, m L =1.37 × 10 −21 g. For NPs after the exchange reaction mass losses below and above 260 °C were treated separately. The number of alkyl ligands in Ag@C 12 H 25 SH: 520. The number of alkyl ligands in Ag@L: 240. The number of L ligands in Ag@L: 260. Numerical calculations The numerical calculations were performed with an in-house code introduced in ref. 66 . For the metal parameters, the data of Johnson and Christy with a size correction for the imaginary part were used; this is necessary as soon as the particles are much smaller than the wavelength, that is, especially when they are small relative to the mean free path of the electrons in a metal. To simulate a reasonable chunk of matter a structure of three shifted layers of 17 times 17 silver spheres with radius 2.35 nm, as it was found in the TEM measurements, was considered for the extinction spectra of the Lm phase. This was sufficient to let all interesting properties converge. The layers were separated by 8.6 nm and the spheres were placed on a square grid with a period of 6.1 nm according to the SAXRD and TEM measurements. To simulate the Iso phase, all spheres of the previous structure were shifted by a random amount in a random direction to negate the long-range order of the structure and to achieve a nearest-neighbour distance of 7.2 nm. To get the effective material properties of the Iso phase the Clausius–Mossotti relation was used. Therefore, the polarizability of a single silver sphere was computed and the filling factor as extracted from the SAXRD measurements was used to calculate the effective permittivity. We used a second code capable of calculating the reflection and transmission coefficients of three layers of an infinitely extended lattice, which is a good representation of the lamellar structure. Again the interparticle and interlayer distances from the SAXRD and TEM measurements of the Lm phase were used. From these reflection and transmission coefficients the effective permittivity was calculated. To cross-check the methods, we also used the Clausius–Mossotti relation using a filling factor corresponding to the Lm phase and a very good agreement was found as is shown in Supplementary Fig. 13 . Bandwidths of the ENZ properties of the Ag@L material were retrieved from identifying the spectral range where Re( ε eff ) values are in between −1.0 and 1.0 ( Supplementary Fig. 9 ). On the basis of the retrieved values of effective permittivity, real and imaginary parts of refractive index were calculated, which allowed us to calculate FOM defined as Re( n eff )/2 Im( n eff ). Ellipsometric measurements For the ellipsometric measurements, a thin film of Ag@L NPs in toluene/chloroform ( v / v =9:1) mixture was spin casted onto two types of substrates: boron-doped silicone wafer substrate cut along [911] plane (CEMAT SILICONE S.A.) and alumina. The substrates with the NP film were then heated to 120 °C and cooled slowly to room temperature in the manner corresponding to samples prepared for SAXRD measurements, to assure the Lm structure of the aggregate. Then, the thicknesses of the samples were measured using AFM, showing relatively low height variance. Amplitude (Psi) and phase (Delta) of the complex reflectance ratio were measured for wavelengths from 400 to 800 nm with a 2-nm step, at 70°, 65° and 60° angle of incidence. Data were fitted using SpectraRay II software package (SENTECH Instruments GmbH) by minimizing the square root of variance. To fit the substrates software built-in functions for Si and Al covered with Al 2 O 3 were used, achieving parameters in agreement with the literature values. For the purpose of fitting the acquired ellipsometric data (amplitude and phase of reflected light versus light wavelength, Supplementary Fig. 11 ), we rely on a complex function for the effective permittivity based on two assumptions—that the material is made from small, spherical particles made of silver (properties of which can be reflected by a permittivity function for Ag that is built in the software) embedded into an organic matter with aromatic moieties (properties thereof are reflected by a harmonic oscillator with free parameters). It should be noted that similar results were obtained when using an effective medium approach with Bruggeman analysis, approximating the medium as a mixture of aromatic molecules (reflected by an oscillator) and silver (reflected by the built-in permittivity for Ag). Imaginary part of ε inf was set to 0 and not fitted. We have taken care to find the global minimum for fitting the data by large, random changes of the function parameter values. A sample result characteristic to a whole set of samples is given in Supplementary Fig. 11 (Si substrate). AFM measurement of film thickness for the same sample (ca. 100 nm) is given in Supplementary Fig. 10 . The data taken for different samples exhibit similar characteristics with an anomaly occurring below 500 nm, but slightly differing depending on the film thickness, roughness and uniformity of the sample. The mean square error of the fitting shown in Supplementary Fig. 11 is 1.1. How to cite this article: Lewandowski, W. et al . Dynamically self-assembled silver nanoparticles as a thermally tunable metamaterial. Nat. Commun . 6:6590 doi: 10.1038/ncomms7590 (2015).